A magnetic non-reciprocal isolator for broadband terahertz operation A Faraday isolator is an electromagnetic non-reciprocal device, a key element in photonics. It is required to shield electromagnetic sources against the effect of back-reflected light, as well as to limit the detrimental effect of back-propagating spontaneous emissions. A common isolator variant, the circulator, is widely used to obtain a complete separation between forward- and backward-propagating waves, thus enabling the realization of a desired transfer function in reflection only. Here we demonstrate a non-reciprocal terahertz Faraday isolator, operating on a bandwidth exceeding one decade of frequency, a necessary requirement to achieve isolation with the (few-cycle) pulses generated by broadband sources. The exploited medium allows a broadband rotation, up to 194°/T, obtained using a SrFe 12 O 19 terahertz-transparent permanent magnet. This in turn enables the design of a stand-alone complete terahertz isolator without resorting to an external magnetic field bias, as opposed to all the optical isolators realized so far. While a general non-vacuum material is an electromagnetic reflective/absorptive attenuator by nature, its phase transfer function is normally quite hard to manipulate. However, having control over the phase has always been quite important. Phase retarders (PRs), that is, devices that induce a phase shift on the transmitted or reflected wave, are fundamental parts of any communication or electromagnetic processing system. They come at the core of many complex devices like filters, delay lines, modulators, isolators, switches and circulators. Although a transparent birefringent crystal (that is, a crystal whose refractive index varies with both the light polarization and the direction of propagation) naturally induces a phase shift between the two distinct field components, this linear field–matter interaction is, by definition, reciprocal. In other words, the reflected polarized beams retrieve their original polarization states as they travel back through the same birefringent medium. Field–matter interactions with media subjected to magnetic fields can exhibit breaking of such symmetry. Over a century ago, Lord Rayleigh described a one-way transmission system based on the mechanism of Faraday rotation [1] . Linearly polarized light can be decomposed into two counter-rotating circular eigenmodes of equal amplitude. In Faraday rotators, the sign of the phase shift between the circular eigenmodes is reversed when the wavevector is reversed. As this is accompanied by a reversal of the propagation coordinates, both the forward and the backward propagation induce the same phase retardation (that is, with the same sign), leading to an output polarization state different from the input one in the reflected wave. Consequently, if the rotation angle is adjusted to 45° and the rotating medium is placed between two specifically aligned polarizers, light propagates in one direction only. Such non-reciprocity finds its application in many fundamental systems. In the microwave regime, isolators, gyrators and circulators are basic examples of non-reciprocal elements that have been vital parts of microwave systems over the past half century [2] , [3] , [4] , [5] . Looking at the optical frequencies, isolators are extremely popular in the realization of both laser devices and photonic circuits. Unidirectional propagation is a typical requirement in fibre laser sources or in amplification chains, as shown for instance in [6] , [7] , [8] , [9] . At the upper end of the gigahertz band, isolators have already been crucial components in the operation and testing of important systems such as free electron lasers [10] (240 GHz) and in the Plank telescope [11] (320 GHz). The available isolation frequency lines and the highest achievable isolation frequency set a limit on the range of systems to which this device can be applied [12] . Recent advances in terahertz generation and detection have allowed the exploitation of waves covering the whole terahertz spectrum. Tunable narrowband [13] and ultra broadband sources [14] , [15] , [16] , [17] , [18] as well as detectors [19] start now to be available. Such sources find a wide range of applications extending from triggering nonlinear phenomena [20] , [21] , [22] , [23] , [24] to linear applications such as imaging [25] , [26] , communications [27] and spectroscopy of chemicals and explosives [28] , [29] . In all those cases, experiments require broadband or tunable sources, which can easily cover more than a spectral decade. While sources and detectors can handle broadband pulses, supporting devices (such as modulators, isolators, filters and so on) remain the actual bandwidth bottleneck. In the light of this work, an isolator or, generally speaking, a non-reciprocal PR is a fundamental element, for example to pave the way to terahertz lasers and amplifiers [30] . We would like to stress that such a constraint is remarkably important in the terahertz region owing to the large relative bandwidths exploited, whereas for example in optics, spectral widths are commonly small fractions of the carrier wave frequency. Not surprisingly, owing to these severe constraints, and in spite of its enormous importance, a terahertz isolator has not been realized so far. Here, we demonstrate that strontium iron oxide (SrFe 12 O 19 ) magnets, commercially available ferrites, can be used as ultra wideband adjustable non-reciprocal PRs at terahertz frequencies. By controlling the induced retardation, we demonstrate a fully functional terahertz isolator, operating over one decade in frequency. Structural and magnetic properties Faraday rotation at terahertz frequencies has been demonstrated at room temperature in both solid [31] , [32] and liquid [33] samples. However, in comparison, our PR has three main advantages towards the realization of an isolation device. First, the induced Faraday rotation is weakly sensitive to frequency in the terahertz band. This originates mainly from the fact that strontium ferrites exhibit a ferromagnetic resonance around 50–60 GHz (depending on the applied magnetic field) [34] , thus far below the terahertz regime. This allows for a very low-dispersive operation. Second, although ferrites generally exhibit magnetic properties similar to those of conducting ferromagnets, their conductivities are in general very low. Isolators require PRs where significant polarization rotation is obtained upon propagation. This directly correlates the maximum achievable rotation to the inherent losses. Terahertz low-loss media are, therefore, fundamental for practical devices. Finally, SrFe 12 O 19 falls under the general class of permanent (hard) magnets, that is, it retains its magnetic state when the external magnetizing field is removed. Hence, contrary to their optical counterparts, external magnets are not required to sustain the isolator operation. A schematic diagram of the sample parameters is shown in Fig. 1a along with the rotation characterization setup and the terahertz polarizations conventions used in this work. Our sample is a 25.4-mm-diameter, 3-mm-thick disk that can be magnetized in any direction. The phase structure of SrFe 12 O 19 has been verified using X-ray diffraction (XRD). The saturation magnetization of the sample was found to be 360 kA m −1 using a vibrating sample magnetometer (VSM) (see Methods for details). 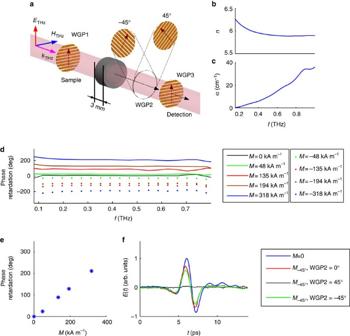Figure 1: Sample characterization. (a) Schematic diagram of a three-polarizer setup to measure the phase retardation induced by the magnetization state of the sample. WGP1 and WGP3 are set to 0° (that is, the grid lines are orthogonal to the terahertz electric field polarization, leading to maximum transmission). WGP2 is oriented to 45° and −45°, respectively. (b) Refractive index and (c) absorption coefficient of SrFe12O19in the frequency range of 0.15–1 THz. Standard THz-TDS spectroscopy was employed to obtain the transfer function of the sample, from which the complex dielectric function was retrieved. (d) Spectral dependence of the phase retardation for different magnetization levels. In order to confirm the non-reciprocity of the device, we reversed the magnetic field direction. Consistently, the sign of the measured rotation changed (dotted plots). (e) Remanence magnetization dependence (linearity check) of the phase retardation measured at 0.35 THz. (f) Transmitted terahertz pulse for specific cases: non-magnetized sample (blue line) and −45°-magnetized sample for three orientations of the analyser WGP2 (red, black and green lines). Figure 1: Sample characterization. ( a ) Schematic diagram of a three-polarizer setup to measure the phase retardation induced by the magnetization state of the sample. WGP1 and WGP3 are set to 0° (that is, the grid lines are orthogonal to the terahertz electric field polarization, leading to maximum transmission). WGP2 is oriented to 45° and −45°, respectively. ( b ) Refractive index and ( c ) absorption coefficient of SrFe 12 O 19 in the frequency range of 0.15–1 THz. Standard THz-TDS spectroscopy was employed to obtain the transfer function of the sample, from which the complex dielectric function was retrieved. ( d ) Spectral dependence of the phase retardation for different magnetization levels. In order to confirm the non-reciprocity of the device, we reversed the magnetic field direction. Consistently, the sign of the measured rotation changed (dotted plots). ( e ) Remanence magnetization dependence (linearity check) of the phase retardation measured at 0.35 THz. ( f ) Transmitted terahertz pulse for specific cases: non-magnetized sample (blue line) and −45°-magnetized sample for three orientations of the analyser WGP2 (red, black and green lines). Full size image Dielectric and terahertz properties Measurements of the complex dielectric function, that is, the spectroscopy measurements, presented in this work have been performed using a standard terahertz time-domain spectroscopy (THz-TDS) setup [35] . Terahertz pulses were generated via optical rectification in a ZnTe crystal illuminated by femtosecond Ti:sapphire laser pulses (130-fs long at a repetition rate of 1 kHz) having a wavelength centred around 800 nm. The detection has been performed by means of the electro-optical sampling technique using a second ZnTe crystal. Note that we used a relatively thick (3 mm) sample and that isolation characterization requires the field to pass twice through the rotator. This limits our transparency window to 0.08–0.8 THz. However, as shown in the next paragraphs, the device exhibits high rotation and the isolation can be achieved with~1 mm-thick samples. As shown in Fig. 1a , the terahertz electric and magnetic fields are assumed to oscillate along the y and x axis, respectively, whereas the terahertz wave wavevector lies in the out-of-plane (sample normal) z direction. In order to retrieve the complex refractive index of the sample, we determined the field transfer function T ( ω ) defined as: where E s ( ω ) and E r ( ω ) are the Fourier transforms of the temporal field functions detected when the terahertz propagates through the sample and when the sample is removed (reference), respectively. The calculated refractive index and the absorption coefficient are shown in Fig. 1b for the case of a non-magnetized sample. Under such a condition, the medium does not exhibit any significant anisotropy and the residual medium magnetization does not contribute to the terahertz phase delay used to calculate the dielectric function. To demagnetize the sample, we applied a reverse magnetic field in order to remove the net out-of-plane magnetization in the entire region illuminated by the terahertz field. It should be noted, however, that part of the absorption shown in Fig. 1c comes from domain wall losses that are reduced upon magnetization of the sample, that is, following the alignment of the magnetic domains. Phase retardation characterization Starting with a non-magnetized state, the sample was permanently magnetized along the terahertz propagation axis by applying gradually and incrementally an external magnetizing field before each measurement. The out-of-plane remanence magnetization at each measurement was estimated by probing the magnetic induction at a specific distance from the sample surface. Subsequently, it was calibrated against the saturation magnetization (see Methods for details). The magnetization state was also found to be stable over time after the applied magnetic field was removed. The measurement of the polarization state of the material at a given magnetization state was performed by means of an ellipsometry setup, made up of three wire-grid polarizers (WGP1; WGP2; and WGP3), as shown in Fig. 1a . We assume that at 0°, the wire-grid polarizers are transmissive for the vertically polarized terahertz electric field, that is, their wire comb is horizontally aligned. We note that this condition corresponds to the maximum transmitted signal. WGP1 and WGP3 were set to 0° to ensure a vertical linear polarization for both the generated and detected signals. By adjusting the rotation of WGP2 to 45° and −45° from the maximum transmission position, respectively, we probed two orthogonal polarization states that were mapped directly to the circular radiation eigenmodes [33] , [36] . Both Faraday polarization rotation (equivalent to half the phase retardation value) and ellipticity were readily found for different magnetization levels. While the transmitted field exhibited a negligible ellipticity, significant retardation reaching 210° was measured for a magnetizing induction B of 540 mT ( Fig. 1d ). Such a field corresponds to a remenant magnetization of 318 kA m −1 as obtained from the VSM measurements. We determined the magneto-optical Verdet constant, defined as the Faraday rotation normalized to the magnetization strength and the sample thickness d , to have a broadband value of v≈ 1.53 × 10 3 rad T −1 m −1 , in turn leading to a figure of merit (FOM)=rotation angle × e − αd of 1.376, 0.620 and 0.096 rad calculated for the maximum rotation angle at 0.2, 0.3 and 0.5 THz, respectively. In the case of a non-magnetized sample, a negligible rotation (<6°) was measured. This value is consistent with the accuracy of the ellipsometry measurement and with the small residual magnetization always induced by the edges of the sample. Reversing the direction of the applied field leads to a reversal of the retardation sign. This confirms the non-reciprocity of the device and distinguishes it from regular non-magnetic ones. The retardation was also found to be flat over the considered frequency range. To check the magnetic field dependence of the retardation, we show the phase retardation at 0.35 THz for different magnetization ( M ) levels ( Fig. 1e ). As expected, within the experimental accuracy, the retardation is linearly proportional to the internal magnetization. The data provided in Fig. 1d show that the sample can induce non-reciprocal adjustable phase retardation, up to 210°, for a propagation length of 3 mm. As a direct application, we demonstrate here a fully functional broadband isolator. The required phase retardation for isolation purposes can be obtained by simply magnetizing the sample to obtain a polarization rotation of 45° upon propagation through it ( Fig. 1f ). Owing to its non-reciprocity, a reflected wave back-propagating through the isolator encounters a similar phase shift that adds up to a total of a 90° polarization rotation, that is, the reflected polarization is crossed with respect to the original wave. If a 0°-aligned polarizer is placed before the isolator, such a back-propagating crossed wave is eliminated and does not reach the source or the other preceding parts in the system. Using the data obtained from our measurements, we applied a magnetizing field corresponding to a remanence magnetization of 135 kA m −1 to induce the required 45° rotation. The functionality of the proposed terahertz isolator has been tested using the backward-waves characterization setup shown in Fig. 2 , where a flat mirror is normally placed after the sample to allow for the terahertz wave to back-propagate through the same sample. Two polarizers are used in this configuration following the typical Faraday isolator design: WGP4 is set to 0° and WGP5 is set to 45°. 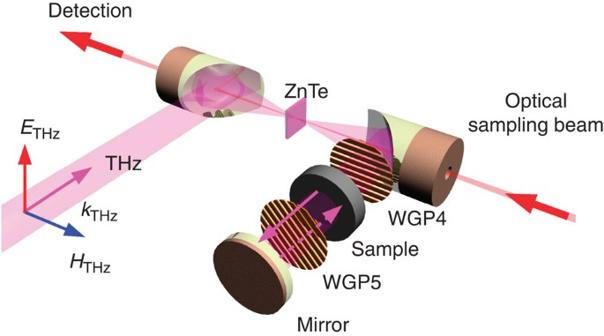Figure 2: Isolator characterization setup. A two-polarizer (WGP4 and WGP5) configuration is employed. WGP4 is set to 0° to ensure a vertical polarization of both the generated and detected signals. Figure 2: Isolator characterization setup. A two-polarizer (WGP4 and WGP5) configuration is employed. WGP4 is set to 0° to ensure a vertical polarization of both the generated and detected signals. 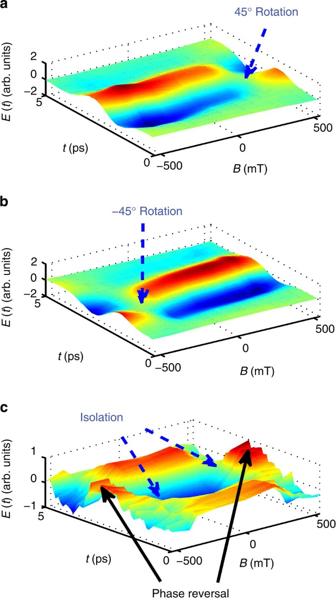Figure 3: Rotations and phase retardation mapping. Transmitted terahertz wave when WGP2 is aligned to (a) −45° and (b) 45°, respectively. Rotation is shown to change sign when the direction of the applied magnetic field is reversed. (c) Back-reflected wave for different magnetizing fields. The isolation and phase reversal points (where 90° and 180° rotations are induced in the reflected wave, respectively) are marked in the plot. Full size image Figure 3 shows the mapping of the rotation induced upon forward transmission through the sample ( Fig. 3a ) in the ellipsometry setup, as well as the total retardation accumulated by the wave when it is back-reflected towards the source ( Fig. 3c ) in this isolator configuration (but now, without WGP5). The isolation points correspond to a 90° rotation in the back-reflected wave. It is noteworthy to point out that as the magnetization is further increased, the back-reflected wave can be completely phase reversed as demonstrated in the figure. Figure 3: Rotations and phase retardation mapping. Transmitted terahertz wave when WGP2 is aligned to ( a ) −45° and ( b ) 45°, respectively. Rotation is shown to change sign when the direction of the applied magnetic field is reversed. ( c ) Back-reflected wave for different magnetizing fields. The isolation and phase reversal points (where 90° and 180° rotations are induced in the reflected wave, respectively) are marked in the plot. Full size image Owing to non-reciprocity, the whole retardation process is flipped when the sign of the magnetic field is reversed. To estimate the isolation depth, two time traces extracted from Fig. 3c at 0 and 135 kA m −1 of remanence magnetization are shown in Fig. 4 . When the sample is not magnetized, the back-reflected field is completely transmitted when WGP5 is not present or it is placed oriented at 0°. This demonstrates that no polarization rotation occurs. The polarizer induces a small delay as it can be readily deduced by simply comparing the two plots. Conversely, when the medium is magnetized, no terahertz radiation is detected and complete isolation (within the sensitivity of our detection) is obtained when WGP5 is not present or when is placed and oriented at 45°. As the isolation is not achieved for any other orientation of WGP5, this confirms that the rotator exhibits a 45° polarization rotation within the experimental accuracy. 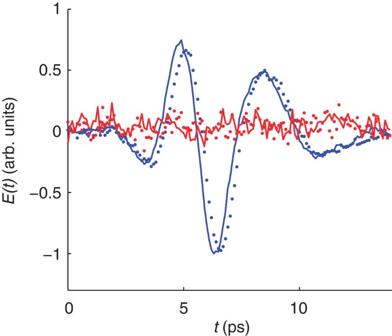Figure 4: Isolator characterization. The back-reflected terahertz pulse was measured using the isolator setup. The comparison is made between a 45°-magnetized sample (the isolator case, shown in red) and an unmagnetized one (shown in blue). Solid/dotted lines refer to the cases where WPG5 was removed/placed, respectively. Figure 4: Isolator characterization. The back-reflected terahertz pulse was measured using the isolator setup. The comparison is made between a 45°-magnetized sample (the isolator case, shown in red) and an unmagnetized one (shown in blue). Solid/dotted lines refer to the cases where WPG5 was removed/placed, respectively. Full size image In conclusion, we introduced an adjustable non-reciprocal PR operating at terahertz frequencies. By controlling the retardation, we designed and experimentally showed a broadband terahertz isolator extending over a frequency decade. The general non-reciprocal phase retardation presented here can be applied to non-reciprocal field displacement, coupling and rotation. We believe that our results will pave the way for a new class of terahertz devices exploiting magnetic field-induced non-reciprocity, either as stand-alone components or integrated with other reciprocal systems, as well as for the realization of terahertz lasers and amplifiers. Structural characterization The sample phase was characterized using the XRD technique, which is an analytical technique that can be used to reveal the chemical and physical composition of materials. As X-ray wavelengths are comparable to the interatomic distances, measurement of the diffracted X-ray gives information about the crystal structure. A typical diffractometer records the intensity of the diffracted waves at different angles (XRD θ– 2 θ spectrum). The angular spectrum is characteristic of a specific crystal structure and is used to identify and confirm the material phase. We carried out the characterization using a Rigaku (D/MAX-2200/PC) X-ray diffractometer with a Cu K-alpha radiation line using the JCPDS file no. 33-1340. 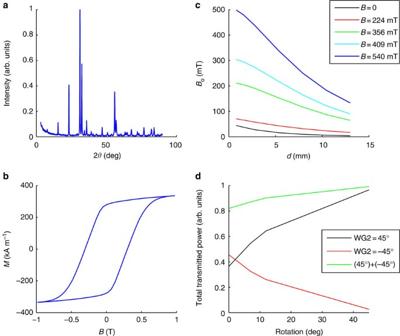Figure 5: Magnetic medium characterization. (a) Measured XRD spectrum depicting the crystalline phase of SrFe12O19. (b) Hysteresis curve obtained from VSM measurements. (c) Induction field at specific points from the sample surface measured at different magnetization stages. (d) The total transmitted power versus the induced rotation for two orthogonal orientations of WG2. In green, the sum of the recorded power for the two conditions is plotted. Figure 5a shows the XRD θ– 2 θ spectrum, which confirms the SrFe 12 O 19 crystalline phase. Figure 5: Magnetic medium characterization. ( a ) Measured XRD spectrum depicting the crystalline phase of SrFe 12 O 19 . ( b ) Hysteresis curve obtained from VSM measurements. ( c ) Induction field at specific points from the sample surface measured at different magnetization stages. ( d ) The total transmitted power versus the induced rotation for two orthogonal orientations of WG2. In green, the sum of the recorded power for the two conditions is plotted. Full size image Magnetic medium characterization The magnetic medium was characterized via the measurement of the hysteresis curve (magnetization state M versus the applied induction field B ) using a Lakeshore VSM (model 7400) at room temperature. Figure 5b shows the hysteresis behaviour of the sample where the saturation magnetization was found to be 360 kA m −1 . In order to estimate the remanence magnetization after each magnetization stage, we measured the induction field intensity ( B 0 ) at specific distances ( d ) from the sample and calibrated it against the remanence at saturation (obtained from the hysteresis curve). The decay of the magnetic induction with the distance from the sample is shown in Fig. 5c . Terahertz spectroscopy and calculation of dielectric function THz-TDS is a standard technique for material characterization in the terahertz regime. Owing to the coherent nature of the available terahertz detection techniques, a time trace of the terahertz field amplitude can be recorded. Its Fourier transform reveals both the amplitude and the phase of the terahertz pulse spectrum. This allows for the complete characterization of the terahertz radiation and of the material-induced effects, thus providing an important spectroscopic tool for extracting the material properties in the terahertz regime. As a direct application here, we used THz-TDS to calculate the complex dielectric function of our sample. The technique is based on the measurement of the transmitted terahertz pulse through the sample and the corresponding reference when the sample is removed. The transmission amplitude was then calculated using Equation 1, from which both the refractive index and material absorption coefficient were subsequently retrieved. Losses and frequency dependences In this section, we would like to highlight the effect of the two main non-idealities of a real isolator, indeed affecting our realization in the terahertz band: inherent losses and frequency dependence of the retardation. In ferrites, magnetic domain walls in the unmagnetized state induce transmission losses. The latter are reduced when the sample gets magnetized and the domain walls vanish. For example, although Fig. 1c shows specific (and relatively high) losses for an unmagnetized sample, the power transmission of the sample increases by 22% as we magnetize it to obtain a rotation of 45° (required by the isolator), see Fig. 5d . Most importantly, in addition to SrFe 12 O 19 being relatively transparent in the terahertz regime, this material does not exhibit significant circular dichroism when magnetized along the direction of propagation. This means that the right and left circularly polarized modes in the retarder undergo the same attenuation. Said otherwise, the rotation—and hence the isolation properties—are unaffected by the losses. In the light of this, we would like to stress that the critical criterion in the choice of a material for an isolator is the independence of the phase retardation from the frequency. Concerning the feasibility of an isolation device at terahertz wavelengths, it is shown in ref. 37 that frequency-independent rotation is, in general, expected above the material magnetic resonance. The latter is conveniently located in the sub-terahertz regime for many ferrites. In addition, ferrites exhibit low group velocity dispersion in the terahertz domain, a property that is always considered an advantage when dealing with the propagation of short (broadband) pulses. We could not characterize the retardation above 1 THz owing to the limited signal to noise ratio of our detection system and our relatively large sample thickness. However, we expect that by using the thickness required to get a 45° polarization rotation at the magnetization saturation (~ 1 mm), the isolator transparency window will enlarge consistently. How to cite this article: Shalaby, M. et al . A magnetic non-reciprocal isolator for broadband terahertz operation Nat. Commun. 4:1558 doi: 10.1038/ncomms2572 (2013).